Transcriptional read-through of the long non-coding RNASVALKAgoverns plant cold acclimation Most DNA in the genomes of higher organisms does not encode proteins, yet much is transcribed by RNA polymerase II (RNAPII) into long non-coding RNAs (lncRNAs). The biological significance of most lncRNAs is largely unclear. Here, we identify a lncRNA ( SVALKA ) in a cold-sensitive region of the Arabidopsis genome. Mutations in SVALKA affect CBF1 expression and freezing tolerance. RNAPII read-through transcription of SVALKA results in a cryptic lncRNA overlapping CBF1 on the antisense strand, termed asCBF1 . Our molecular dissection reveals that CBF1 is suppressed by RNAPII collision stemming from the SVALKA-asCBF1 lncRNA cascade. The SVALKA-asCBF1 cascade provides a mechanism to tightly control CBF1 expression and timing that could be exploited to maximize freezing tolerance with mitigated fitness costs. Our results provide a compelling example of local gene regulation by lncRNA transcription having a profound impact on the ability of plants to appropriately acclimate to challenging environmental conditions. RNA Polymerase II (RNAPII) transcription in genomes results in the production of many long non-coding RNAs (lncRNAs) [1] . The functional significance of resulting lncRNA molecules is actively debated even though biological roles have been identified for an increasing number of examples [2] , [3] , [4] . Expression of lncRNAs is remarkably specific to the environmental condition, tissue or cell type, arguing for roles of lncRNAs in regulation [5] , [6] , [7] . In addition to functions carried out by lncRNA molecules, the process of transcribing non-coding DNA sequences can by itself be regulatory in many systems [8] , [9] . Non-coding DNA regions in genomes can therefore affect gene expression by different mechanisms that need to be resolved experimentally. Sessile organisms respond to changing environmental conditions by the regulation of gene expression. Early events in the Arabidopsis cold response include rapid transcriptional up-regulation of the intron-less C-repeat/dehydration-responsive element binding factors (CBFs) [10] , [11] . The CBFs are highly conserved transcription factors that promote cold tolerance in many plant species and are often arranged in a single cluster [12] . CBF expression during cold exposure activates downstream COLD REGULATED (COR) genes that promote freezing tolerance by adjusting the physiological and biochemical properties of plant cell interiors [13] , [14] , [15] . Intriguingly, constitutive CBF expression increases cold tolerance but is also associated with fitness penalties [16] , [17] , [18] , [19] . For example, over-expression of CBF1 results in increased tolerance to freezing temperatures, but also severely reduces biomass [20] . Therefore, the expression of the endogenous CBF1 gene is characterized by a transient peak of maximal expression during cold acclimation [11] . The negative fitness costs of both increased and decreased CBF expression highlight the importance of their tight regulation, yet the specific mechanisms that tightly control CBF expression during the early response to cold are not fully understood. The plant response following long exposure to cold temperatures is associated with numerous lncRNAs that associate with the FLOWERING LOCUS C ( FLC ) gene. The antisense lncRNA COOLAIR is induced after 2 weeks of cold, and initiates chromatin repression of the FLC gene [2] , [21] . Full FLC silencing is aided by polycomb repressive complex recruitment by the intron-derived lncRNA COLDAIR and reinforced by the promoter derived lncRNA COLDWRAP [22] . This cold-triggered cascade of lncRNAs establishes long-lasting and stable repression of the FLC gene and serves as a paradigm for gene repression by lncRNAs [23] . However, it is currently unresolved if early responses to cold temperatures in plants are mediated by lncRNAs. Here, we map transcriptional start sites in Arabidopsis during early responses to cold temperatures. We identify a cascade of two lncRNAs that fine-tune the expression of the CBF1 gene. Transcriptional read-through of the lncRNA SVALKA results in the expression of a cryptic antisense CBF1 lncRNA ( asCBF1 ). asCBF1 transcription results in RNAPII collision to limit the expression of full-length CBF1 . This work extends the biological roles of lncRNAs during cold acclimation and it provides an elegant mechanism that achieves rapid dynamic regulation of environmentally sensitive gene expression. Identification of the lncRNA SVALKA To identify transcription initiation events that respond to cold temperature in Arabidopsis , we performed transcription start site (TSS)-sequencing(TSS-seq) [24] , [25] . We obtained 184 million raw reads from two biological replicates at 22 °C and two biological replicates at 3 h of 4 °C. From these, we called 14250 TSS clusters. Our analyses revealed 489 down-regulated and 1404 up-regulated TSSs in response to 3 h at 4 °C (Fig. 1a , Supplementary Data 1 , Supplementary Data 2 ). Most differentially used TSSs were located in promoter regions corresponding to changed promoter usage in fluctuating environments. Of the up-regulated genes (±200 bp of the major TSS), the CBF genes were upregulated 100–400 fold making the CBF genomic region by far the most cold-responsive region in the genome (Fig. 1b ). Interestingly, we detected a cold-responsive lncRNA, transcribed on the antisense strand between CBF3 and CBF1 (Fig. 1c ) that we named SVALKA ( SVK , for short). We found two TSSs by Rapid Amplification of cDNA Ends (RACE) that corresponded to the peaks observed with TSS-seq (Fig. 1d ). Our 3′RACE analysis also supported the existence of alternative SVK isoforms. 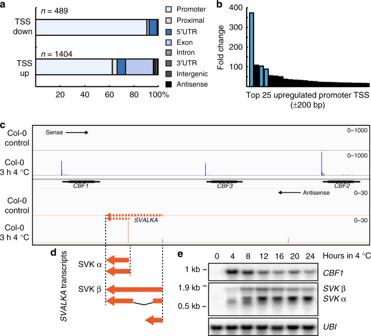Fig. 1 Transcription Start Site (TSS) sequencing in Col-0 after 3 h of exposure to 4 °C identified the long non-coding RNA,SVALKA.aDifferentially expressed TSS after cold exposure in Col-0. A total of 1893 TSS changed their expression significantly (p< 0.05). Of these, 489 were down-regulated while 1404 were up-regulated. The TSS were classified according to their position relative to  gene bodies . The majority of differentially expressed TSS were found in or around promoters.bActivity of up-regulated promoters after cold exposure identities theCBFgenes (indicated in blue bars) as highly up-regulated. Graph represents the fold change of the top 25 up-regulated promoters in Col-0 after cold exposure.cScreenshot of theCBFgenomic region and the identified TSS. The upper panel shows the sense TSS-seq reads direction (blue) and clear TSS can be found for the threeCBFgenes. The lower panel shows the TSS-seq reads in antisense direction (orange) where a group of cold-induced TSS was identified in the intergenic region betweenCBF1andCBF3.dSummary of 3′- and 5′-RACE ofSVALKA. Two clusters of capped TSS were found forSVALKA, a distal TSS centered around 2360 bp and a proximal TSS centered around 1386 bp in respect to the translation start ofCBF1. A cluster of polyadenylation sites were found 846–897 bp in respect to the translation start ofCBF1. The plethora ofSVALKAtranscripts includes a spliced isoform with a splice site from 1386 to 2113 bp in respect to the translation start ofCBF1.eRNA levels ofCBF1andSVALKAduring a time course of cold exposure of Col-0. WhileCBF1transiently is upregulated early in the cold response,SVALKAresponds later and its expression is anti-correlated to senseCBF1.UBIis used as a loading control. Experiments were done with three biological replicates showing similar results. Uncropped blots can be found in the Source Data file 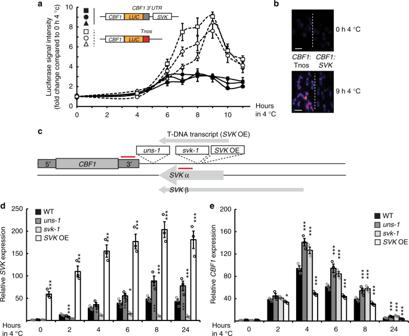Fig. 2 Characterization of the long non-coding RNA,SVALKA.aLUCIFERASE (LUC) activity of two differentCBF1-LUCconstructs. White markers indicate three independent transformants of a construct whereLUCexpression is driven by theCBF1promoter and terminated by the TNOSterminator (CBF1:TNOS). Black markers indicate three independent transformants of constructs whereLUCexpression is driven by the CBF1 promoter with the endogenousCBF1terminator and fullSVALKAsequence (CBF1:SVK). The CBF1:SVK lines showed a decreased LUC activity following cold exposure compared to the CBF1:TNOS) lines. LUC activity was measured as average pixel intensity of at least 5 seedlings for each time point. Markers represent mean with standard deviation. Source data are provided as a Source Data file.bRepresentative images of lines in control conditions and after 9 h of cold exposure for the two LUC constructs. Scale bar represents 1 cm.cGraphical representation of the insertion positions of the T-DNA lines used in this study. The qPCR probes are indicated with red and used in (d) and (e). See Supplementary Figure5for additional information on the insertion mutants.d,eRelativeSVK(d) andCBF1(e) expression determined by RT-qPCR in WT and mutants that effectSVKfollowing exposure to cold. Bars represent mean (black: WT, dark grey:uns-1, light grey:svk-1, white:SVK OE, ±SEM) from three biological replicates (rings). The relative level ofSVKandCBF1transcripts were normalized to the level in WT in control conditions. Statistically significant differences between means were determined with Student’st-test (*p< 0.05, ***p< 0.001). Source data are provided as a Source Data file Notably, we detected no transcript overlapping the downstream CBF1-3′UTR (Supplementary Figure 1 , Supplementary Figure 2 ). 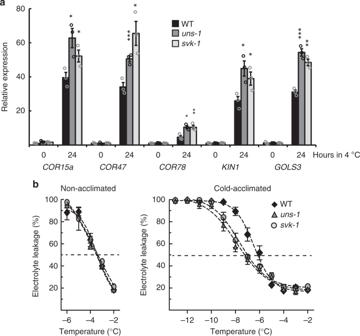Fig. 3 Mutants that affectSVKshow increased freezing tolerance.aRelative level of different cold-responsive transcripts in control and after 24 h of cold exposure in WT,svk-1anduns-1determined by RT-qPCR. Bars represent mean (black: WT, dark grey:uns-1, light grey:svk-1, ±SEM) from three biological replicates (rings). The relative level of theCORtranscripts were normalized to the level in WT in control conditions. Statistically significant differences were determined with Student’st-test (*p< 0.05, **p< 0.01, ***p< 0.001). Source data are provided as a Source Data file.bElectrolyte leakage in non-acclimated (left panel) and cold-acclimated (right panel) WT (black),svk-1(light grey) anduns-1(dark grey) plants. Leaf discs of each genotype were in contact with deionized water in a test tube and exposed to −2 °C for 1 h followed by a decreased temperature at a rate of 2 °C/h. Samples were taken out at the indicated temperatures and the solution in the tubes was measured for electrolytes. Subsequently, each tube was submersed in liquid nitrogen allowed to thaw and measured again for electrolytes. Each marker represents the mean electrolyte leakage (electrolyte content before exposure to liquid nitrogen/total electrolyte content) after freezing test compared to the total electrolyte content (±standard deviation) from at least three biological replicates. Source data are provided as a Source Data file RT-qPCR revealed that more SVK is generated from the CBF1- proximal promoter than from the distal promoter (Supplementary Figure 3 ), consistent with TSS-seq analyses. A time series of cold exposure (4 °C) with samples taken every 4 h revealed the expression pattern of SVK and CBF1 (Fig. 1e ). CBF1 expression peaked at 4 h followed by a decrease that reached a relatively stable level after 12–16 h, a pattern in congruence with earlier studies [26] . In contrast, SVK showed gradual increase in expression from 4 h to reach a stable maximum level after 12–16 h. Fig. 1 Transcription Start Site (TSS) sequencing in Col-0 after 3 h of exposure to 4 °C identified the long non-coding RNA, SVALKA . a Differentially expressed TSS after cold exposure in Col-0. A total of 1893 TSS changed their expression significantly ( p < 0.05). Of these, 489 were down-regulated while 1404 were up-regulated. The TSS were classified according to their position relative to  gene bodies . The majority of differentially expressed TSS were found in or around promoters. b Activity of up-regulated promoters after cold exposure identities the CBF genes (indicated in blue bars) as highly up-regulated. Graph represents the fold change of the top 25 up-regulated promoters in Col-0 after cold exposure. c Screenshot of the CBF genomic region and the identified TSS. The upper panel shows the sense TSS-seq reads direction (blue) and clear TSS can be found for the three CBF genes. The lower panel shows the TSS-seq reads in antisense direction (orange) where a group of cold-induced TSS was identified in the intergenic region between CBF1 and CBF3 . d Summary of 3′- and 5′-RACE of SVALKA . Two clusters of capped TSS were found for SVALKA , a distal TSS centered around 2360 bp and a proximal TSS centered around 1386 bp in respect to the translation start of CBF1 . A cluster of polyadenylation sites were found 846–897 bp in respect to the translation start of CBF1 . The plethora of SVALKA transcripts includes a spliced isoform with a splice site from 1386 to 2113 bp in respect to the translation start of CBF1 . e RNA levels of CBF1 and SVALKA during a time course of cold exposure of Col-0. While CBF1 transiently is upregulated early in the cold response, SVALKA responds later and its expression is anti-correlated to sense CBF1 . UBI is used as a loading control. Experiments were done with three biological replicates showing similar results. Uncropped blots can be found in the Source Data file Full size image SVK represses CBF1 and promotes cold acclimation The anti-correlation between CBF1 and SVK and their genomic proximity suggested that SVK could be involved in CBF1 repression. To test this, we constructed two distinct LUCIFERASE (LUC) reporter lines of CBF1 with different termination sequences. We expected any repressive role of SVK to be present in the lines with endogenous 3′-sequences ( CBF1 : SVK) . In contrast, we expected effects of SVK to be absent in the lines with the terminator sequences of the NOPALINE SYNTHASE (NOS) gene that shows low antisense transcription [4] ( CBF1 :T NOS ). We subjected three independent lines from each construct to 4 °C for 0–12 h and subsequently measured LUC activity (Fig. 2a, b ). The three CBF1 :T NOS lines showed increased LUC activity compared to the CBF1 : SVK lines. These data demonstrated that SVK represses LUC activity. We wanted to confirm these findings by measuring antisense transcription from the 3′-end of the LUC constructs. Therefore, we designed a qPCR based strategy to measure antisense transcription that may be initiated from the endogenous CBF1–3′-UTR or the T NOS terminator [4] . 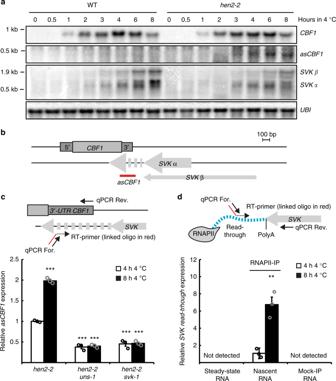Fig. 4 SVALKAtranscription mediates transcription activity antisense toCBF1.aRepresentative Northern blot of a cold exposure time series of Col-0 (WT) andhen2-2. The probe used forasCBF1is shown inb. Blots were repeated with three biological replicates with similar results.UBIis used as loading control. Uncropped blots can be found in the Source Data file.bGraphical representation of theCBF1-SVKgenomic region. The probe forasCBF1is shown in red. RT was done with an oligo-linked primer to ensure strand-specificity and generated cDNA was used inc.cRT-qPCR ofasCBF1after cold exposure inhen2-2and the double mutants,hen2-2uns-1,andhen2-2svk-1. The RT-primer and the qPCR primers are shown in the graphical representation above the graph. Bars represent mean (white: 4 h 4 °C, black: 8 h 4 °C, ±SEM) from three biological replicates (rings). The relative level ofasCBF1was normalized to the level inhen2-2after 4 h of 4 °C. Statistically significant differences were determined with Student’st-test (***p< 0.001). Source data are provided as a Source Data file.d) RT-qPCR ofSVKread-through transcripts. Hundred nanograms of RNA from an RNAPII-IP (i.e. RNA attached to RNAPII) or total RNA was converted to cDNA with an oligo-linked primer. The RT-primer and qPCR primers used can be seen in the graphical representation above the graph. The RT-primer annealed to a sequence downstream of the PolyA signal ofSVK. A read-through transcript can be detected in the nascent RNA samples with an increased expression after 8 h of cold exposure. No signal could be seen in the Mock-IP or total RNA sample. Each bar represents the mean (white: 4 h 4 °C, black: 8 h 4 °C, ±SEM) from three biological replicates (rings). The relative level of read-through transcripts was normalized to the level in the nascent sample after 4 h of 4 °C. Statistically significant differences were determined with Student’st-test (***p< 0.001). Source data are provided as a Source Data file We detected antisense transcription from the T NOS sequence in two independent CBF1 :T NOS lines (Supplementary Figure 4 ). However, antisense transcription from T NOS was not cold-responsive, arguing against a cold-induced effect of LUC expression. In contrast, we detected cold-induced antisense akin to SVALKA transcription from the endogenous CBF1 −3′-UTR in the CBF1:SVK lines (Supplementary Figure 4 ). These data suggest that cold-induced antisense transcription could be involved in regulating endogenous CBF1 expression. Fig. 2 Characterization of the long non-coding RNA, SVALKA . a LUCIFERASE (LUC) activity of two different CBF1 - LUC constructs. White markers indicate three independent transformants of a construct where LUC expression is driven by the CBF1 promoter and terminated by the T NOS terminator (CBF1:T NOS ). Black markers indicate three independent transformants of constructs where LUC expression is driven by the CBF1 promoter with the endogenous CBF1 terminator and full SVALKA sequence (CBF1:SVK). The CBF1:SVK lines showed a decreased LUC activity following cold exposure compared to the CBF1:T NOS ) lines. LUC activity was measured as average pixel intensity of at least 5 seedlings for each time point. Markers represent mean with standard deviation. Source data are provided as a Source Data file. b Representative images of lines in control conditions and after 9 h of cold exposure for the two LUC constructs. Scale bar represents 1 cm. c Graphical representation of the insertion positions of the T-DNA lines used in this study. The qPCR probes are indicated with red and used in ( d ) and ( e ). 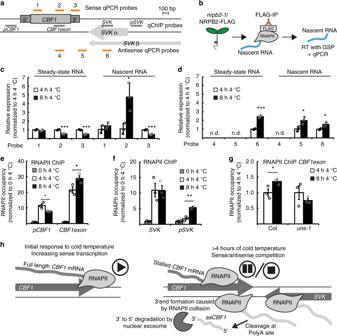Fig. 5 Antisense transcription toCBF1results in stalling mRNA transcription at the 3′-end ofCBF1.aGraphical representation of the sense and antisense qPCR probes used incandd. RT was done with an oligo-linked primer to ensure strand-specificity. qChIP probes used ine–gare indicated with a dashed black line.bGraphical visualization of the RNAPII-IP to isolate nascent RNA.c–d) RT-qPCR with the sense probes (1–3,c) and with the antisense probes (4–6,d). All probes are shown ina. Nascent RNA was compared to a total RNA preparation (steady-state level of RNA). Bars represent mean (white: 4 h 4 °C, black: 8 h 4 °C, ±SEM) from three biological replicates (rings). The relative level of transcripts was normalized to the level at 4 h 4 °C. Statistically significant differences between 4 and 8 h of 4 °C were determined with Student’s t-test (*p< 0.05, ***p< 0.001). Source data are provided as a Source Data file.e–gqChIP of total RNAPII along theCBF1genomic region following cold exposure in WT (e), of theSVKgenomic region in WT (f) and of theCBF1transcription unit in WT and theuns-1mutant following 4 and 8 h of 4 °C (g). The location of promoter (pCBF1),CBF1exon, the promoter (pSVK) and SVK probes can be seen ina. Bars represent the mean of three biological replicates (grey: 0 h 4 °C, white: 4 h 4 °C, black: 8 h 4 °C, ±SEM) and are normalized to the level at 0 h 4 °C. Statistically significant differences were determined with Student’st-test (*p< 0.05, **p< 0.01, ***p< 0.001). Source data are provided as a Source Data file.hMechanistic model of how transcription ofSVKrepresses senseCBF1transcription. Initially during cold exposure,SVKis not expressed and senseCBF1can be transcribed without hindrance (left panel).CBF1expression peaks after 4 h of cold exposure. Simultaneously, expression of the lncRNASVKis increased in the antisense direction ofCBF1(right panel). Read-through transcription ofSVKresults in transcription antisense to the 3′-end ofCBF1and an increase of RNAPII occupancy on both strands. The intensification of transcribing polymerases in both directions creates RNAPII collision and stalling ofCBF1sense transcription. The outcome of the collision is that fewer RNAPII complexes reach the end of theCBF1sense transcription unit and a decrease of full-lengthCBF1mRNA See Supplementary Figure 5 for additional information on the insertion mutants. d , e Relative SVK ( d ) and CBF1 ( e ) expression determined by RT-qPCR in WT and mutants that effect SVK following exposure to cold. Bars represent mean (black: WT, dark grey: uns-1 , light grey: svk-1 , white: SVK OE , ±SEM) from three biological replicates (rings). The relative level of SVK and CBF1 transcripts were normalized to the level in WT in control conditions. Statistically significant differences between means were determined with Student’s t -test (* p < 0.05, *** p < 0.001). Source data are provided as a Source Data file Full size image We next characterized Arabidopsis Transfer DNA (T-DNA) lines to further dissect the function of the CBF1 3′-region. T-DNA lines insert large sequences of DNA (often 4–5 kb) in the Arabidopsis genome that disrupt the genomic context at the insertion site [27] . We isolated three informative T-DNA insertion mutants: (1) a line that disrupted SVK ( svk-1 ), (2) a line that increased the distance of SVK transcription from CBF1 ( uncoupling svalka-1, uns-1 ), and (3) a line that showed SVK over-expression ( SVK OE ) (Fig. 2c , Supplementary Figure 2 , 5 ). The SVK over-expression originates from strong promoters within the T-DNA that continued over the insertion border (Supplementary Figure 5a-b ). We could not detect any other T-DNA driven transcription in the svk- 1 or uns-1 mutants (Supplementary Figure 5c-d ). We quantified SVK and CBF1 expression by RT-qPCR. svk-1 showed reduced expression of SVK while the uns-1 mutants showed slightly elevated levels of SVK compared to wild-type. As expected, the SVK OE mutant showed greatly increased level of SVK (Fig. 2d ). Interestingly, we detected CBF1 mis-regulation in all three mutants (Fig. 2e ). The combination of high level of SVK expression and increased CBF1 expression in uns-1 compared to wild-type argues against a trans-acting function for the SVK lncRNA (Fig. 2d, e ). In this mutant, SVK is expressed 4–5 kb away (compared to 110 bp for wild-type) from CBF1 but CBF1 expression is still increased compared to wild-type. Both the uns-1 and svk-1 mutants showed an increase of CBF1 expression in response to cold exposure, while the SVK OE mutant lead to decreased CBF1 levels, supporting the notion that SVK plays a repressive role on CBF1 mRNA levels. We could not see any effect on the neighboring CBF3 and CBF2 genes (Supplementary Figure 6 ). Increased CBF1 levels in the uns-1 and the svk-1 mutants lead to greater induction of CBF -activated COR genes (Fig. 3a ). These findings suggested that SVK transcription could have a biologically important role and affect cold acclimation and freezing tolerance. We conducted an electrolyte leakage test of wild-type, svk-1 and uns-1 plants to test the role of SVK in freezing tolerance (Fig. 3b ). In this test, leaf discs of non-acclimated and cold-acclimated plants are in contact with water and exposed to decreasing freezing temperatures and measured for leakage of electrolytes (i.e., plasma membrane disruption). Surviving cells keep their electrolytes within the cell. Therefore, measuring electrolyte leakage is a measurement of how well the cells can survive freezing temperatures [28] . Cold-acclimated svk-1 and uns-1 showed a higher freezing tolerance compared to wild type. Wild-type plants showed an electrolyte leakage of 50% at −6.5 °C (±0.2 °C, 95% CI) compared to svk-1 (−7.7 °C, ±0.2 °C) and uns-1 (−7.9 °C, ±0.3 °C). The increase in freezing tolerance is remarkable and is similar to that of the myb15 mutant, a transcription factor that directly suppresses CBF expression [29] . Together, our findings suggest that the genomic region encoding SVK represses cold-induced CBF1 expression and has a biologically relevant effect on cold acclimation and freezing tolerance in Arabidopsis . Fig. 3 Mutants that affect SVK show increased freezing tolerance. a Relative level of different cold-responsive transcripts in control and after 24 h of cold exposure in WT, svk-1 and uns-1 determined by RT-qPCR. Bars represent mean (black: WT, dark grey: uns-1 , light grey: svk-1 , ±SEM) from three biological replicates (rings). The relative level of the COR transcripts were normalized to the level in WT in control conditions. Statistically significant differences were determined with Student’s t -test (* p < 0.05, ** p < 0.01, *** p < 0.001). Source data are provided as a Source Data file. b Electrolyte leakage in non-acclimated (left panel) and cold-acclimated (right panel) WT (black), svk-1 (light grey) and uns-1 (dark grey) plants. Leaf discs of each genotype were in contact with deionized water in a test tube and exposed to −2 °C for 1 h followed by a decreased temperature at a rate of 2 °C/h. Samples were taken out at the indicated temperatures and the solution in the tubes was measured for electrolytes. Subsequently, each tube was submersed in liquid nitrogen allowed to thaw and measured again for electrolytes. Each marker represents the mean electrolyte leakage (electrolyte content before exposure to liquid nitrogen/total electrolyte content) after freezing test compared to the total electrolyte content (±standard deviation) from at least three biological replicates. Source data are provided as a Source Data file Full size image Read-through transcription of SVK results in asCBF1 To better understand the mechanism of SVK repression, we revisited the effects of the uns-1 insertion. uns-1 is inserted downstream of SVK yet results in equivalent cold-related defects compared to svk-1 . A possible explanation for the effects seen in the svk-1 and uns-1 mutants would be that read-through transcription of CBF1 is reduced by the T-DNA insertions that may increase the stability of the CBF1 mRNA. The Arabidopsis 5′−3′ exonuclease XRN3 is associated with the removal of uncapped nuclear transcripts that are expected for read-through transcripts derived from RNAPII termination [30] . Consistently, we find increased CBF1 read-through transcription in the xrn3–3 mutant (Supplementary Figure 7 ). However, we could not detect decreased CBF1 read-through in the svk-1 and uns-1 mutants, arguing against increased mRNA stability linked to increased transcriptional termination efficiency in these mutants (Supplementary Figure 7 ). Another possibility that could reconcile our findings would be if SVK was promoting transcription of a cryptic antisense transcript into the CBF1 gene body, since such a transcript would be disrupted in uns-1 and svk-1 . To test this hypothesis, we carefully examined the presence of an antisense transcript mapping to the 3′-UTR of CBF1 (Fig. 4a, b ). HEN2 is part of the nucleoplasmic 3′ to 5′ exosome responsible for degrading many types of non-coding RNAPII transcripts [31] . We used a high resolution time series of cold exposed samples of wild type and hen2-2 to enable the detection of cryptic antisense transcripts. A CBF1 antisense transcript ( asCBF1 ) corresponding to roughly 250 nt was detectable in the hen2-2 mutant, yet not in the wild type (Fig. 4a , Supplementary Figure 8a ). asCBF1 was also detected in additional mutants disrupting the nuclear exosome (Supplementary Figure 8b ). However, we could not detect asCBF1 in the sop1-5 ( suppressor of pas2 ) mutant that have an increase of a subset of HEN2-dependent degradation targets [32] or the trl-1 mutant, which is disrupted for TRL1 (TRF4/5-like), a factor involved in 3′-processing of rRNA in the nucleolus [33] (Supplementary Figure 8b ). Together, these results suggest asCBF1 transcript is a nucleoplasmic exosome target with expression levels correlated to SVK . The size of asCBF1 suggests it is either a SVK read-through transcript that is cleaved at the poly-(A) signal or a new transcription initiation event. To confirm that asCBF1 depends on SVK transcription, we crossed the svk-1 and uns-1 mutants to hen2-2 (Fig. 4c ). In both double mutants, the asCBF1 RNA was lost, confirming that asCBF1 transcription depends on SVK . Fig. 4 SVALKA transcription mediates transcription activity antisense to CBF1 . a Representative Northern blot of a cold exposure time series of Col-0 (WT) and hen2-2 . The probe used for asCBF1 is shown in b . Blots were repeated with three biological replicates with similar results. UBI is used as loading control. Uncropped blots can be found in the Source Data file. b Graphical representation of the CBF1-SVK genomic region. The probe for asCBF1 is shown in red. RT was done with an oligo-linked primer to ensure strand-specificity and generated cDNA was used in c . c RT-qPCR of asCBF1 after cold exposure in hen2-2 and the double mutants, hen2-2uns-1, and hen2-2svk-1 . The RT-primer and the qPCR primers are shown in the graphical representation above the graph. Bars represent mean (white: 4 h 4 °C, black: 8 h 4 °C, ±SEM) from three biological replicates (rings). The relative level of asCBF1 was normalized to the level in hen2-2 after 4 h of 4 °C. Statistically significant differences were determined with Student’s t -test (*** p < 0.001). Source data are provided as a Source Data file. d ) RT-qPCR of SVK read-through transcripts. Hundred nanograms of RNA from an RNAPII-IP (i.e. RNA attached to RNAPII) or total RNA was converted to cDNA with an oligo-linked primer. The RT-primer and qPCR primers used can be seen in the graphical representation above the graph. The RT-primer annealed to a sequence downstream of the PolyA signal of SVK . A read-through transcript can be detected in the nascent RNA samples with an increased expression after 8 h of cold exposure. No signal could be seen in the Mock-IP or total RNA sample. Each bar represents the mean (white: 4 h 4 °C, black: 8 h 4 °C, ±SEM) from three biological replicates (rings). The relative level of read-through transcripts was normalized to the level in the nascent sample after 4 h of 4 °C. Statistically significant differences were determined with Student’s t -test (*** p < 0.001). Source data are provided as a Source Data file Full size image Transcription in higher eukaryotes occurs beyond the poly-(A) termination signal before nascent transcript cleavage is triggered [34] . Nascent transcript cleavage creates the 3′-end of the full-length mRNA substrate for poly-adenylation, and a free 5′-end is attacked by 5′ to 3′ exonucleases eliciting transcription termination according to the torpedo model [35] , [36] . To detect any read-through transcription from SVK , we purified RNA associating with RNAPII complexes (Supplementary Figure 9a ). To isolate nascent RNA, we used a stable Arabidopsis line with a FLAG-tagged version of NRPB2 (i.e., the second largest subunit of RNAPII). After IP, NRPB2 co-eluted with NRPB1, confirming that we purified intact RNAPII complexes (Supplementary Figure 9b-d ). Subsequently, we isolated the RNA attached to the purified RNAPII complexes. We profiled this RNA for the presence of SVK transcripts extending into CBF1 as antisense transcripts with qPCR (Fig. 4d ). We detected quantifiable levels of a read-through product after 4 h of cold exposure and increased expression after 8 h in the nascent RNA fraction. Consistent with asCBF1 being a product of read-through following SVK 3′-end formation and cleavage, we could not detect the SVK-asCBF1 read-through transcript in total RNA (i.e. steady state) or in a Mock-IP control samples (i.e. IP with a non-FLAG tagged line). Detection in nuclear exosome mutants and nascent transcript preparation gives asCBF1 characteristics of a cryptic lncRNA that is quickly cleaved and degraded in wild-type. XRN3 is thought to represent the 5′-to-3′ torpedo exonuclease mediating transcriptional termination in Arabidopsis [30] , [36] . However, we did not detect the asCBF1 RNA or CBF1 mRNA mis-regulation in the xrn3-3 mutant (Supplementary Figure 10 ). These data suggest that transcriptional termination of SVK read-through is either XRN3 independent, or the hypomorphic xrn3-3 allele does not disrupt XRN3 function strong enough to detect SVK termination defects. In summary, our findings revealed asCBF1 as a HEN2 -dependent “cryptic” antisense transcript that depends on SVK read-through transcription during cold to repress CBF1 induction. CBF1 expression is limited by RNAPII collision Two molecular mechanisms could explain the observed SVK -mediated effects on CBF1 expression: (1) transcription of asCBF1 activates the siRNA pathway to trigger repression [37] , or (2) the act of asCBF1 transcription itself causes sense/antisense competition and RNAPII collision [38] . To test if siRNA were involved, we performed cold exposure of several different mutants in various siRNA pathways and probed for CBF1 mRNA levels (Supplementary Figure 11a ). All the mutants failed to show increased CBF1 levels (Supplementary Figure 11b ), ruling out the siRNA model. A RNAPII collision model predicts a discrepancy of transcription between the 5′-end and the 3′-end of CBF1 caused by stalled RNAPII transcription complexes in the 3′-end of CBF1 [38] . Our protocol to isolate nascent RNA enabled us to detect strand-specific sites of RNAPII accumulation (i.e., potential pause sites) with RT-qPCR (Fig. 5b , Supplementary Figure 9 ). The 5′-end probe (Probe 1 in Fig. 5c ) showed no significant difference, suggesting that RNAPII occupancy early in CBF1 elongation was indistinguishable between 4 and 8 h of 4 °C. The probe in the 3′-end of the CBF1 exon (Probe 2 in Fig. 5c ) showed that RNAPII occupancy was significantly increased over this region of CBF1 after 8 h compared to 4 h. Intriguingly, the increased RNAPII occupancy at the 3′-end of the CBF1 exon was not detected in the 3′-UTR (Probe 3 in Fig. 5c ). These data are consistent with the collision model that predicts RNAPII complexes are pre-maturely terminated before they have time to fully transcribe a full-length CBF1 transcript. Fig. 5 Antisense transcription to CBF1 results in stalling mRNA transcription at the 3′-end of CBF1 . a Graphical representation of the sense and antisense qPCR probes used in c and d . RT was done with an oligo-linked primer to ensure strand-specificity. qChIP probes used in e – g are indicated with a dashed black line. b Graphical visualization of the RNAPII-IP to isolate nascent RNA. c – d ) RT-qPCR with the sense probes (1–3, c ) and with the antisense probes (4–6, d ). All probes are shown in a . Nascent RNA was compared to a total RNA preparation (steady-state level of RNA). Bars represent mean (white: 4 h 4 °C, black: 8 h 4 °C, ±SEM) from three biological replicates (rings). The relative level of transcripts was normalized to the level at 4 h 4 °C. Statistically significant differences between 4 and 8 h of 4 °C were determined with Student’s t-test (* p < 0.05, *** p < 0.001). Source data are provided as a Source Data file. e – g qChIP of total RNAPII along the CBF1 genomic region following cold exposure in WT ( e ), of the SVK genomic region in WT ( f ) and of the CBF1 transcription unit in WT and the uns-1 mutant following 4 and 8 h of 4 °C ( g ). The location of promoter ( pCBF1 ), CBF1 exon, the promoter ( pSVK ) and SVK probes can be seen in a . Bars represent the mean of three biological replicates (grey: 0 h 4 °C, white: 4 h 4 °C, black: 8 h 4 °C, ±SEM) and are normalized to the level at 0 h 4 °C. Statistically significant differences were determined with Student’s t -test (* p < 0.05, ** p < 0.01, *** p < 0.001). Source data are provided as a Source Data file. h Mechanistic model of how transcription of SVK represses sense CBF1 transcription. Initially during cold exposure, SVK is not expressed and sense CBF1 can be transcribed without hindrance (left panel). CBF1 expression peaks after 4 h of cold exposure. Simultaneously, expression of the lncRNA SVK is increased in the antisense direction of CBF1 (right panel). Read-through transcription of SVK results in transcription antisense to the 3′-end of CBF1 and an increase of RNAPII occupancy on both strands. The intensification of transcribing polymerases in both directions creates RNAPII collision and stalling of CBF1 sense transcription. The outcome of the collision is that fewer RNAPII complexes reach the end of the CBF1 sense transcription unit and a decrease of full-length CBF1 mRNA Full size image The 3′-UTR probe assays the steady state level of full-length CBF1 mRNA (Fig. 2e ). The steady state CBF1 RNA levels after 4 and 8 h of cold exposure showed lower levels of CBF1 transcripts containing the middle (probe 2 in Fig. 5c ) and the end (probe 3 in Fig. 5c ) than the beginning of CBF1 (probe 1 in Fig. 5c ). These data confirm that the major decrease after 8 h of cold exposure in full-length CBF1 mRNA levels relate to differences in the 3′-end. In agreement with these results, we could detect high amounts of pre-maturely terminated CBF1 when sense transcripts are probed in the 5′-end compared to the 3′-end with Northern blot (Supplementary Figure 12 ). This effect was exaggerated in the hen2-2 mutant, suggesting that many pre-terminated CBF1 events are rapidly degraded by the nuclear exosome. Probes for antisense transcripts of SVK showed an increasing RNAPII occupancy over the SVK transcription unit following longer exposure to cold (Probe 6 in Fig. 5d ). We detected SVK read-through transcripts in the nascent fraction (Probe 5 in Fig. 5d ). No products were detected with the probe further downstream (Probe 4 in Fig. 5d ). These data support that RNAPII complexes are terminated before transcription reaches further into the CBF1 exon. This is also consistent with the size of the asCBF1 transcript (Fig. 4a ). We complemented these results with total RNAPII quantitative Chromatin Immuno-Precipitation (qChIP) analyses following exposure to 4 °C. Reminiscent of the results from analyzing nascent transcripts, we detected a higher RNAPII occupancy over the CBF1 exon after 8 h compared to 4 h of 4 °C. In contrast, the probe at the promoter of CBF1 ( pCBF1 in Fig. 5a–e ) showed a decrease of RNAPII occupancy after 8 h. These results strongly suggest that RNAPII complexes are stalled in the 3′-end of CBF1 since full-length CBF1 mRNA levels decrease after 8 h compared to 4 h of cold exposure (Figs 1e , 5c ). qChIP probes for SVK showed higher use of the SVK promoter following cold exposure that was also seen for the SVK transcription unit (Fig. 5f ). Another prediction of the collision model is that increased RNAPII occupancy over the CBF1 exon in wild-type should be abolished in the uns-1 mutant, since no collision would occur due to the absence of asCBF1 transcription. Our hypothesis was tested and confirmed by qChIP for total RNAPII over the CBF1 exon in wild type and uns-1 since no increase of RNAPII occupancy was observed in the uns-1 mutant (Fig. 5g ). Collectively, these results imply the presence of stalled RNAPII complexes over the 3′-end of CBF1 that were correlated with increased asCBF1 expression. In conclusion, our results showed that read-through of a lncRNA triggers head-to-head RNAPII collision over the CBF1 gene body leading to regulated termination of CBF1 transcription and a decrease of full-length CBF1 mRNA levels (Fig. 5h ). This study illustrates how lncRNA read-through transcription limits peak expression of gene expression to promote an appropriate response to environmental change. Environmental change alters RNAPII transcription in genomes so that organisms can adequately respond to new conditions [5] , [39] . These transcriptional responses include high RNAPII activity in non-coding regions, resulting in lncRNA transcription. On the one hand, lncRNA molecules may provide function, for example through riboswitch regulation [40] , [41] . On the other hand, the process of lncRNA transcription by RNAPII can affect the regulation of gene expression in the vicinity of target genes [42] . A curious result of widespread lncRNA transcription is that genes are often transcribed on both DNA strands, resulting in mRNA from the sense strand, and lncRNA from the antisense strand [43] . Antisense transcription is detected in many genomes, and genome-wide analyses suggest that these phenomena can be either positively or negatively correlated with the corresponding sense transcript [44] . The positive correlations between sense and antisense expression represent a puzzling conundrum, as this relationship poses the question of how two converging RNAPII enzymes transcribing the same DNA can move past each other [38] . Sense and antisense transcription pairs on cell population level have been resolved as binary expression states for the individual transcripts at single-cell level [45] . Perhaps alternative expression states of sense or antisense lncRNA transcription in individual cells offers an explanation for why examples of gene repression by RNAPII collision are relatively rare. Overall, antisense transcription appears to be a common strategy to affect gene repression [44] . Our study uncovers how the interplay between two lncRNAs limits the production of maximal mRNA levels of the Arabidopsis CBF1 gene by an RNAPII collision mechanism in the 3′-end of CBF1 . Cold-induced transcription initiation in the CBF locus triggers expression of a cascade of antisense transcripts that fine-tunes the level of CBF1 mRNA, thereby representing a negative feedback required for plants to appropriately acclimate to low temperatures. The identification of interplay between a stable lncRNA SVALKA and a cryptic lncRNA asCBF1 acting together in gene repression represents an important aspect of our study. The cryptic lncRNA asCBF1 is detectable after 6 h of cold treatment in nuclear exosome mutant backgrounds. asCBF1 is likely representative of additional lncRNAs with regulatory roles that are challenging to study owing to their cryptic and environmental specific expression characteristics. Our findings of multiple lncRNAs acting together is in line with recent findings suggesting a coordinated effect of multiple lncRNAs to regulate meiosis in yeasts [46] , [47] . The combinations of multiple lncRNAs amplify the interfaces with regulatory potential and may increase precision of target regulation. Since asCBF1 results from RNAPII read-through transcription of SVK , our findings highlight the process of transcriptional termination of lncRNAs for regulation. Selective transcriptional termination of the Arabidopsis lncRNA COOLAIR determines FLC expression states by a chromatin-based mechanism [2] . A similar mechanism is more difficult to elucidate in this case due to the relatively small size of the CBF1 gene body (i.e. 946 bp). Moreover, the class of budding yeast stable uncharacterized transcripts (SUTs) with environment-specific expression is characterized by inefficient termination resulting in read-through transcription into neighboring genes. Consistently, regulation of yeast gene expression by read-through transcription of SUTs is well-documented [48] . Extended SUT species link transcripts to create interdependency of loci to achieve coordinated expression changes [43] . The effects of the SVK-asCBF1 circuitry support the idea that cascades of lncRNA transcription provide a mechanism to coordinate local regulation. lncRNA cascades increase the spacing distance between initial lncRNA transcription events and the target gene, in contrast to a straightforward antisense lncRNA. Multiple cascading transcripts provide more room for independent regulatory inputs to achieve precision in regulation. The topology of the Arabidopsis genome is thought to be gene-centric with local gene loops rather than larger topologically associated domains (TADs) [49] , [50] . We would expect extensive co-regulation if sense and antisense lncRNA transcription were part of the same gene loop. Indeed, alternative gene loop formation is triggered by transcription of the lncRNA APOLO to regulate expression of the PINOID gene [51] . Read-through transcription of the lncRNA SVALKA may provide a mechanism to invade and break positive feedback mechanisms reinforcing CBF1 transcription. As lncRNA transcription in yeast and mammalian cells correlate with the boundaries of chromatin domains, roles of lncRNA in communicating regulation across domain boundaries may be common despite differences in genomic topologies [52] , [53] . The entire transcripts in the CBF cluster increase expression in response to short-term cold temperatures [11] . The discovery of the SVK-asCBF1 lncRNA cascade illustrates how transcriptional activation of this region is associated with an inbuilt negative feedback mechanism that limits the timing of maximal CBF1 expression by triggering RNAPII collision. While CBF genes promote freezing tolerance, excess CBF gene expression is associated with fitness penalties [16] , [17] , [18] , [19] . In this regard, the SVK-asCBF1 cascade provides a mechanism to tightly control maximal CBF1 expression and timing that could be exploited to engineer freezing tolerance with mitigated fitness costs. The conservation of CBF gene clusters and their role in promoting plant freezing tolerance potentially suggests that lncRNA cascades equivalent to SVK-asCBF1 could exist in other species. The lncRNA-mediated effects of long-term cold exposure on plant gene expression have been well characterized for the FLC gene [2] , [45] . Our research demonstrates that lncRNAs also mediate the response to short-term and transient cold exposure by timing maximal gene expression. Future research will be needed to investigate if biophysical properties of lncRNA transcription may provide a particularly effective sensor for temperature. Perhaps more likely, lncRNA functions in temperature responses will coincide with the intensity of research efforts addressing this question in plants to prepare for changing climates. In sum, our findings provide a compelling example of functional lncRNA transcription in cells to limit gene induction by triggering RNAPII collisions. Plant materials and growth conditions A. thaliana seedlings were grown on ½ MS + 1% Sucrose plates in long day photoperiod (16 h light/8 h dark) at 22 °C/18 °C unless otherwise stated. For all experiments, Col-0 was used as wild-type background. All newly characterized T-DNA lines in this study were identified at [ http://signal.salk.edu/cgi-bin/tdnaexpress?gene =] and seeds from the lines were ordered from the Nottingham Arabidopsis Stock Centre. Genotypes used in this study can be found in Supplementary Data 3 . For cold treatment, seedlings were grown in control conditions for 10 days (100 μE m −2 s −1 ) and subsequently transferred to 4 °C for indicated times and sampled. Light intensity during cold treatment was approximately 25 μE m −2 s −1 . For freezing tests, plants were grown in short day conditions (8 h light/16 h dark) at 22 °C/18 °C for 6 weeks. Cold acclimation was performed in short day conditions at 4 °C for 4 days prior to freezing test. Cloning and LUC assay Primers for cloning can be found in Supplementary Data 4 . For the CBF1:Tnos construct, a fragment encompassing the CBF1 promoter and gene body (−1903 bp to +639 bp relative to the translation start) was amplified from genomic DNA with Phusion polymerase (Thermo Fisher Scientific, USA) and ligated to the pENTR/D-TOPO vector (Invitrogen, USA). After sequencing to eliminate any cloning errors the pENTR/ CBF1 vector was incubated with pGWB535 vector in a LR reaction. The final vector, pGWB535/CBF1:Tno s was transformed into Col-0 plants using the floral dip method . For the CBF1:SVK construct, a fragment encompassing the SVK promoter and transcription unit (+643 bp to +3410 bp relative to the CBF1 translation start) was amplified from genomic DNA and fused to a CBF1:LUC fragment amplified from pGWB535/CBF1:Tnos . The fused fragment was ligated to pENTR/D-TOPO and sequenced. A LR reaction between pENTR/CBF1:SVK and pGWB501 produced the final vector, PGWB501/CBF1:SVK , which was transformed into Col-0. Transformed seedlings were selected on Hygromycin plates and their progeny (T2 generation) was used for the LUC assay. For detection of LUC, 10 day old seedlings were treated with cold temperature (4 °C). At indicated times 5 µM D-Luciferin (ZellBio, Germany) was sprayed onto seedlings followed by dark incubation for 30–60 min. LUC was detected using a CCD camera and pixel intensity was determined in ImageJ. The average pixel intensity from at least five seedlings was used to get a mean value and used for statistical analysis (see Source Data file). RNA extraction, northern analysis, RACE, and RT-qPCR Total RNA was extracted using RNeasy Plant Mini Kit (Qiagen, Germany) according to manufacturer′s instructions. Northern analysis was performed as described with minor modifications [48] . Five to 20 µg of total RNA was separated on a 1.2% agarose gel with formaldehyde and 1xMOPS. Gels were blotted overnight onto a nylon membrane and crosslinked with UV radiation. Probes were made in a PCR reaction by incorporating radioactive dTTP ( 32 P, PerkinElmer, USA) from a DNA probe template. Membranes were exposed to a phosphorimager screen (GE Healthcare, UK) for 1–10 days depending on the expression level of the transcript of interest. Screens were subsequently scanned with a Typhoon scanner (GE Healthcare, UK). RACE experiments were done with a SMARTer RACE 5′/3′ Kit (Takara, Japan) according to manufacturer’s instructions. For RT-qPCR, total RNA was DNase treated with TURBO DNase (Thermo Fisher Scientific, USA) and 1 µg DNase treated RNA was subsequently turned into cDNA as per manufacturer’s instructions with Superscript III (Invitrogen, USA) using random primers, oligo dT or gene specific primers depending on the experiment. Diluted cDNA (1:10) was used in a PCR reaction with GoTaq qPCR Master mix (Promega, USA) and run on a CFX384 Touch instrument (Bio-Rad, USA). Data were processed in CFX manager and exported to Excel (Microsoft, USA) for further analysis. Relative expression was calculated and normalized to at least two internal reference genes. All primers used in this study can be found in Supplementary Data 4 . All uncropped membranes and all source data for graphs can be found in the Source Data file. Electrolyte leakage test Electrolyte leakage test was performed [54] with leaf discs of non-acclimated or cold-acclimated plants in glass tubes with 200 μl of deionized water. The tubes were then transferred to a programmable bath at −2 °C (FP51, Julabo, Germany). After 1 h, ice formation was induced and the temperature was slowly decreased (−2 °C/h). Samples were taken out of the bath at designated temperatures and cooled on ice for an hour followed by 4 °C. When all samples were collected, 1.3 ml of deionized water was added and the tubes were shaken overnight at 4 °C. Electrolyte leakage was measured using a conductivity cell (CDM210, Radiometer, Denmark). To get total ion content, tubes were immersed in liquid nitrogen, thawed, shaken again overnight and measured for conductivity. Electrolyte leakage was determined by comparing the measured conductivity before and after the liquid nitrogen treatment. Data was fitted to a sigmoidal dose-response with GraphPad Prism and can be found in the Source Data file. TSS-seq and bioinformatic analysis The genome-wide distribution of TSSs in wild-type was recently mapped in Arabidopsis using 5′-CAP-sequencing [25] . Here, we extend these analyses to 2-week old cold-treated seedlings (3 h at 4 °C). Five micrograms of DNase-treated total RNA were treated with CIP (NEB) to remove non-capped RNA species. 5′-caps were removed using Cap-Clip (CellScript) to permit ligation of single-stranded rP5_RND adapter to 5′-ends with T4 RNA ligase 1 (NEB). Poly(A)-enriched RNAs were captured with oligo(dT) Dynabeads (Thermo Fisher Scientific) according to manufacturer’s instructions and fragmented in fragmentation buffer (50 mM Tris acetate pH 8.1, 100 mM KOAc, 30 mM MgOA) for 5 mins at 80 °C. First-strand cDNA was generated using SuperScript III (Invitrogen) and random primers following manufacturer’s instructions. Second-strand cDNA was generated with the BioNotI-P5-PET oligo and using Phusion High-Fidelity Polymerase (NEB) as per manufacturer’s instructions. Biotinylated PCR products were captured by streptavidin-coupled Dynabeads (Thermo Fisher Scientific), end repaired with End Repair Enzyme mix (NEB), A-tailed with Klenow fragment exo- (NEB), and ligated to barcoded Illumina compatible adapter using T4 DNA ligase (NEB). Libraries were amplified by PCR, size selected using AMPure XP beads (Beckman Coulter), pooled following quantification by Bioanalyzer, and sequenced in single end mode on the following flowcell: NextSeq® 500/550 High Output Kit v2 (75 cycles) (Illumina). For the bioinformatics, all supplementary code for the data analysis pipelines described below is available at [ https://github.com/Maxim-Ivanov/Kindgren_et_al_2018 ]. The NGS data manipulations were detailed in the 01-Processing_5Cap-Seq_data.sh pipeline. In brief, the custom adapter sequences (ATCTCGTATGCCG) were trimmed from 3′ ends of the 5Cap-Seq (TSS-Seq) reads using Trim Galore v0.4.3. Then 8 nt random barcodes (unique molecular identifiers, or UMIs) were trimmed from 5′ ends of reads and appended to read names using a custom script (UMI_to_Fastq_header.py). The resultant Fastq files were aligned to TAIR10 genome using STAR v2.5.2b in the end-to-end mode [55] . SAM files were sorted and converted to BAM using Samtools v1.7 [56] . Reads overlapping the rRNA, tRNA, snRNA and snoRNA genes (obtained from the Araport11 annotation) were filtered out using Bedtools v2.25.0 [57] . In addition, multimapper reads with MAPQ score below 10 were removed by Samtools. Morever, we filtered out PCR duplicates by analyzing groups of reads sharing the same 5′ genomic position and removing reads with redundant UMIs (this was done using a custom script Deduplicate_BAM_files_on_UMI.py). Finally, stranded Bedgraph files were generated using Bedtools. For visualization in genomic browsers, the forward and reverse Bedgraph files corresponding to the same sample were combined together and normalized to 1 million tags. For the downstream analysis in R environment, the stranded Bedgraph files were filtered for coverage ≥ 2x and ensured to contain only genomic intervals with 1 bp width (Expand_bedGraph_to_single_base_resolution.py). The detection of 5′ tag clusters (TCs) was described in detail in the 02-Calling_5Cap-Seq_TSS.R pipeline. It makes an extensive use of the CAGEfightR package [ https://bioconductor.org/packages/release/bioc/html/CAGEfightR.html ] [58] . Adjacent TSS separated by not more than 20 bp were merged into TSS clusters. The TSS clusters were annotated by intersection with various genomic features which were extracted from the TxDb.Athaliana.BioMart.plantsmart28 package. We used following definitions: proximal [TSS-500bp, TSS-100bp] and promoters [TSS-100bp, TSS + 100 bp]. In addition, TSS were further annotated by genomic location (according to TAIR10 and Araport11): promoter, proximal, 5′UTR, exon, intron, 3′UTR, antisense, or intergenic. In case of conflicting annotations, a single annotation was chosen according to the following hierarchy: intergenic < antisense < intron < exon < 5′UTR < proximal < promoter. Differentially expressed TCs were called using the DESeq2 package. Polymerase II IP and nascent RNA purification Five grams of seedlings from a line where a NRPB2-FLAG construct covers a lethal nrpb2-1 mutation (described in ref. [59] ) were grinded to a fine powder. NRPB2 encodes the second largest subunit of the RNAPII complex and since the FLAG-tagged protein covers a lethal mutation it ensures that all RNAPII complexes in the line contain a tagged NRPB2. RNA that was attached to RNAPII (i.e. actively transcribed RNA) was isolated via a FLAG-IP. Control Western blots that showed the validity of the approach are shown in Supplementary Figure 9. The Mock-IP sample represents an RNA sample obtained via an IP reaction from a line without a FLAG-tagged NRPB2. For Mock-IP 5 g of Col-0 seedlings were used. Fifteen milliliters of ice-cold extraction buffer (20 mM Tris-HCl pH 7.5, 300 mM NaCl, 5 mM MgCl 2 (+5 µl/ml 20% Tween, 1 µl/ml RNAseOUT, 5 µl/ml 1 M DTT, prot. inhibitor tablet (Roche, 1 tablet for 50 ml buffer)) was added to the powder and 660 U of DNase I was subsequently added to the mix. After 20 min on ice, the mixture was put into a centrifuge for 10 min (4 °C, 10,000 g) and the supernatant was recovered. The supernatant was filtered through a 0.45 µm filter and added to Anti-FLAG M2 magnetic beads (Sigma-Aldrich, USA). Supernatant and beads were then incubated on a slowly rotating wheel at 4 °C for 3 h. Beads were washed eight times with extraction buffer and immunoprecipitated polymerase complexes were eluted with 2 mg/ml 3xFLAG peptide (ApexBio, USA) for two times 30 min. Purified polymerase complexes was disrupted and attached RNA was extracted by the miRNeasy Mini Kit (Qiagen, Germany) according to manufacturer’s instructions. Hundred nanogram isolated RNA was used to create cDNA with Superscript III (Invitrogen, USA) and gene specific primers. Western blotting Protein samples were separated on a 4–15% TGX gel (Bio-Rad, USA) and blotted onto a PVDF membrane. Membranes were blocked in 5% milk powder dissolved in PBS. Primary antibody was incubated with membrane overnight at 4 °C. Following morning, membranes were washed in PBS + T two times for 10-min and incubated with secondary antibody (Agilent, USA) for 60 min at room temperature. After three times of 5-min washes in PBS+T proteins were detected with Super-Signal West Pico Chemiluminescent (Thermo Fisher Scientific, USA) and developed with a ChemiDoc MP instrument (Bio-Rad, USA). Following antibodies were used in this study: Monoclonal Anti-FLAG M2 antibody (F3165, Anti-Sigma-Aldrich, USA) and Anti-RBP1 antibody (ab140509, abcam, UK). Uncropped gel pictures can be found in the Source Data file. Quantitative chromatin immunoprecipitation (qChIP) Arabidopsis seedlings were grown for 12 days on 1/2 Murashige and Skoog (MS) plates containing 1% sucrose and supplemented with 0.5% Microagar in climate chambers at 22 °C with a 16 h light/8 h dark cycle. For cold-treatment, seedlings were grown in control conditions for 12 days and subsequently transferred to 4 °C for indicated times. Cold-treated seedlings were quickly harvested at 4 °C. Fixation of control and cold-treated seedlings were performed at room-temperature using 1% formaldehyde/PBS and vacuum infiltration. Fixation was stopped by the addition of glycine. qChIP experiments were performed essentially as described in ref. [60] , with minor modifications. For immunoprecipitations, Protein A magnetic beads (GenScript) and 2 µg of an antibody (Anti-Total RNA polymerase II 8WG16, ab817, abcam, UK) were added to solubilized chromatin. Quantitative analysis was performed on captured DNA by qPCR (Bio-Rad). See Supplementary Data 4 for oligonucleotide sequences. ChIP enrichments were calculated as the ratio of product of interest from IP sample to the corresponding input sample. Error bars represent standard error of the mean resulting from at least three independent replicates. Source data can be found in the Source Data file. Code availability All supplementary code for the data analysis pipelines described is available at [ https://github.com/Maxim-Ivanov/Kindgren_et_al_2018 ].